The impact of free-ranging domestic cats on wildlife of the United States Anthropogenic threats, such as collisions with man-made structures, vehicles, poisoning and predation by domestic pets, combine to kill billions of wildlife annually. Free-ranging domestic cats have been introduced globally and have contributed to multiple wildlife extinctions on islands. The magnitude of mortality they cause in mainland areas remains speculative, with large-scale estimates based on non-systematic analyses and little consideration of scientific data. Here we conduct a systematic review and quantitatively estimate mortality caused by cats in the United States. We estimate that free-ranging domestic cats kill 1.3–4.0 billion birds and 6.3–22.3 billion mammals annually. Un-owned cats, as opposed to owned pets, cause the majority of this mortality. Our findings suggest that free-ranging cats cause substantially greater wildlife mortality than previously thought and are likely the single greatest source of anthropogenic mortality for US birds and mammals. Scientifically sound conservation and policy intervention is needed to reduce this impact. Domestic cats ( Felis catus ) are predators that humans have introduced globally [1] , [2] and that have been listed among the 100 worst non-native invasive species in the world [3] . Free-ranging cats on islands have caused or contributed to 33 (14%) of the modern bird, mammal and reptile extinctions recorded by the International Union for Conservation of Nature (IUCN) Red List [4] . Mounting evidence from three continents indicates that cats can also locally reduce mainland bird and mammal populations [5] , [6] , [7] and cause a substantial proportion of total wildlife mortality [8] , [9] , [10] . Despite these harmful effects, policies for management of free-ranging cat populations and regulation of pet ownership behaviours are dictated by animal welfare issues rather than ecological impacts [11] . Projects to manage free-ranging cats, such as Trap-Neuter-Return (TNR) colonies, are potentially harmful to wildlife populations, but are implemented across the United States without widespread public knowledge, consideration of scientific evidence or the environmental review processes typically required for actions with harmful environmental consequences [11] , [12] . A major reason for the current non-scientific approach to management of free-ranging cats is that total mortality from cat predation is often argued to be negligible compared with other anthropogenic threats, such as collisions with man-made structures and habitat destruction. However, assessing the conservation importance of a mortality source requires identification of which species are being killed (for example, native versus non-native invasive species and rare versus common species) in addition to estimation of total numbers of fatalities. Estimates of annual US bird mortality from predation by all cats, including both owned and un-owned cats, are in the hundreds of millions [13] , [14] (we define un-owned cats to include farm/barn cats, strays that are fed by humans but not granted access to habitations, cats in subsidized colonies and cats that are completely feral). This magnitude would place cats among the top sources of anthropogenic bird mortality; however, window and building collisions have been suggested to cause even greater mortality [15] , [16] , [17] . Existing estimates of mortality from cat predation are speculative and not based on scientific data [13] , [14] , [15] , [16] or, at best, are based on extrapolation of results from a single study [18] . In addition, no large-scale mortality estimates exist for mammals, which form a substantial component of cat diets. We conducted a data-driven systematic review of studies that estimate predation rates of owned and un-owned cats, and estimated the magnitude of bird and mammal mortality caused by all cats across the contiguous United States (all states excluding Alaska and Hawaii). We estimate that free-ranging domestic cats kill 1.3–4.0 billion birds and 6.3–22.3 billion mammals annually, and that un-owned cats cause the majority of this mortality. This magnitude of mortality is far greater than previous estimates of cat predation on wildlife and may exceed all other sources of anthropogenic mortality of US birds and mammals. The magnitude of bird mortality caused by cat predation After excluding studies that did not meet a priori inclusion criteria designed to increase the accuracy of our analysis, we developed probability distributions of predation rates on birds and mammals. We combined predation rate distributions with literature-derived probability distributions for US cat population sizes, and we also accounted for the proportion of owned cats allowed outdoors, the proportion of owned and un-owned cats that hunt, and imperfect detection of owned cats’ prey items. We generated an estimated range of bird and mammal mortality caused by cat predation by incorporating the above distributions—including separate predation rate distributions for owned and un-owned cats—and running 10,000 calculation iterations. We augmented US predation data by incorporating predation rate estimates from other temperate regions ( Supplementary Table S1 ). For birds, we generated three US mortality estimates based on predation data from studies in: (1) the United States, (2) the United States and Europe and (3) the United States, Europe, and other temperate regions (primarily Australia and New Zealand). Owing to a lack of US studies of un-owned cat predation on mammals, we estimated mammal mortality using data groupings 2 and 3. 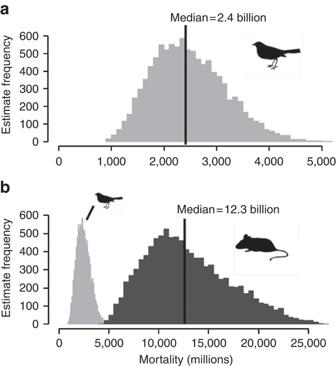Figure 1: Estimates of cat predation on US birds and mammals. (a) Probability distribution of estimated bird mortality caused by all free-ranging cats in mainland areas of the contiguous United States. (b) Probability distribution of estimated mammal mortality caused by all free-ranging cats in mainland areas of the contiguous United States. We based all other probability distributions on US studies (distribution details in Table 1 ; data in Supplementary Table S2 ). Table 1 Probability distributions used for parameters in cat predation model. 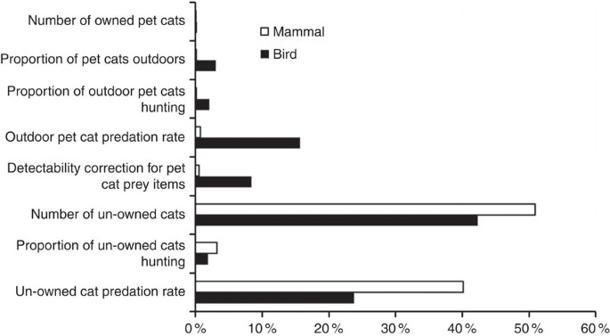Figure 2: Factors explaining uncertainty in estimates of wildlife mortality from cat predation. Amount of variation in estimates of wildlife mortality in the contiguous United States contributed by each parameter in the cat predation model (percentages represent adjustedR2values from multiple regression models). Full size table The three estimates of bird mortality varied moderately, with a 19% difference among median estimates ( Table 2 ). We focus interpretation on the estimate generated using US and European predation data because it is the lowest value. Furthermore, this estimate is more likely to be representative of the US than the estimate based on incorporation of data from Australia and New Zealand, where the wildlife fauna and climate are less similar to the United States. We estimate that cats in the contiguous United States annually kill between 1.3 and 4.0 billion birds (median=2.4 billion) ( Fig. 1a ), with ∼ 69% of this mortality caused by un-owned cats. The predation estimate for un-owned cats was higher primarily due to predation rates by this group averaging three times greater than rates for owned cats. Table 2 Median estimates of annual wildlife mortality caused by cat predation in the contiguous United States. Full size table Figure 1: Estimates of cat predation on US birds and mammals. ( a ) Probability distribution of estimated bird mortality caused by all free-ranging cats in mainland areas of the contiguous United States. ( b ) Probability distribution of estimated mammal mortality caused by all free-ranging cats in mainland areas of the contiguous United States. Full size image The magnitude of mammal mortality caused by cat predation Our estimate of mammal mortality was robust to the choice of predation data as evidenced by a 1.6% difference between the two median estimates ( Table 2 ). We focus interpretation on the lower estimate, which was based on United States and European predation data and US values of other parameters. We estimate annual mammal mortality in the contiguous United States at between 6.3 and 22.3 billion (median=12.3 billion) ( Fig. 1b ) with 89% of this mortality caused by un-owned cats. The estimate that incorporated European data (but not data from Australia and New Zealand) may be slightly lower because wildlife across much of Europe were historically exposed to predation by a similarly-sized wild cat ( Felis sylvestris ) and, therefore, may be less naive to predation by domestic cats. However, it is unlikely that European wildlife have fully adapted to the unusually high densities of domestic cats in much of this continent [9] . Factors explaining estimate uncertainty For both birds and mammals, sensitivity analyses indicated that un-owned cat parameters explained the greatest variation in total mortality estimates ( Fig. 2 ). Un-owned cat population size explained the greatest variation in mortality estimates (42% for birds and 51% for mammals), and the un-owned cat predation rate explained the second greatest variation (24% for birds and 40% for mammals). The only other parameters that explained >5% of variation in mortality estimates were the owned cat predation rate on birds (16%) and the correction factor for imperfect detection of owned cats’ prey items (8%). Figure 2: Factors explaining uncertainty in estimates of wildlife mortality from cat predation. Amount of variation in estimates of wildlife mortality in the contiguous United States contributed by each parameter in the cat predation model (percentages represent adjusted R 2 values from multiple regression models). Full size image Our estimate of bird mortality far exceeds any previously estimated US figure for cats [13] , [14] , [16] , as well as estimates for any other direct source of anthropogenic mortality, including collisions with windows, buildings, communication towers, vehicles and pesticide poisoning [13] , [15] , [16] , [17] , [18] , [19] , [20] , [21] . Systematic reviews like ours, which includes protocol formulation, a data search strategy, data inclusion criteria, data extraction and formal quantitative analyses [22] , are scarce for other anthropogenic mortality sources. [21] Increased rigour of mortality estimates should be a high priority and will allow increased comparability of mortality sources [23] . Nonetheless, no estimates of any other anthropogenic mortality source approach the value we calculated for cat predation, and our estimate is the first for cats to be based on rigorous data-driven methods. Notably, we excluded high local predation rates and used assumptions that led to minimum predation rate estimates for un-owned cats; therefore, actual numbers of birds killed may be even greater than our estimates. Free-roaming cats in the United States may also have a substantial impact on reptiles and amphibians. However, US studies of cat predation on these taxa are scarce. To generate a first approximation of US predation rates on reptiles and amphibians, we used the same model of cat predation along with estimates of cat predation rates on these taxa from studies in Europe, Australia and New Zealand. We estimate that between 228 and 871 million reptiles (median=478 million) and between 86 and 320 million amphibians (median=173 million) could be killed by cats in the contiguous United States each year. Reptile and amphibian populations, and, therefore, cat predation rates, may differ between the regions where we gathered predation data for these taxa and the United States. Furthermore, reptiles and amphibians are unavailable as prey during winter across much of the United States. Additional research is needed to clarify impacts of cats on US herpetofauna, especially given numerous anthropogenic stressors that threaten their populations (for example, climate change, habitat loss and infectious diseases) and documented extinctions of reptiles and amphibians due to cat predation in other regions [4] , [24] . The exceptionally high estimate of mammal mortality from cat predation is supported by individual US studies that illustrate high annual predation rates by individual un-owned cats in excess of 200 mammals per year [6] , [25] , [26] , [27] , [28] and the consistent finding that cats preferentially depredate mammals over other taxa ( Supplementary Table S1 ). Even with a lower yearly predation rate of 100 mammals per cat, annual mortality would range from 3–8 billion mammals just for un-owned cats, based on a population estimate of between 30 and 80 million un-owned cats. This estimated level of mortality could exceed any other direct source of anthropogenic mortality for small mammals; however, we are unaware of studies that have systematically quantified direct anthropogenic mortality of small terrestrial mammals across large scales. Native species make up the majority of the birds preyed upon by cats. On average, only 33% of bird prey items identified to species were non-native species in 10 studies with 438 specimens of 58 species ( Supplementary Table S3 ). For mammals, patterns of predation on native and non-native species are less clear and appear to vary by landscape type. In densely populated urban areas where native small mammals are less common, non-native species of rats and mice can make up a substantial component of mammalian prey [29] . However, studies of mammals in suburban and rural areas found that 75–100% of mammalian prey were native mice, shrews, voles, squirrels and rabbits [26] , [30] , [31] . Further research of mammals is needed to clarify patterns of predation by both owned and un-owned cats on native and non-native mammals, and across different landscape types. Sensitivity analyses indicate that additional research of un-owned cats will continue to improve precision of mortality estimates. Our finding that un-owned cat population size and predation rate explained the greatest variation in mortality estimates reflects the current lack of knowledge about un-owned cats. No precise estimate of the un-owned cat population exists for the United States because obtaining such an estimate is cost prohibitive, and feral un-owned cats are wary of humans and tend to be solitary outside of urban areas. In addition, human subsidized colonies of un-owned cats are maintained without widespread public knowledge. For example, in Washington DC alone there are >300 managed colonies of un-owned cats and an unknown number of unmanaged colonies. Population size estimates can be improved by incorporating observations of free-ranging cats into a wildlife mortality reporting database [23] . Context for the population impact of a mortality source depends on comparing mortality estimates to estimates of population abundance of individual species. However, continental-scale estimates of wildlife population abundance are uncertain due to spatio-temporal variation in numbers. For mammals, clarification of the population impacts of cat predation is hindered by the absence of nationwide population estimates. For all North American land birds, the group of species most susceptible to mainland cat predation ( Supplementary Table S3 ), existing estimates range from 10–20 billion individuals in North America [32] . A lack of detail about relative proportions of different bird species killed by cats and spatio-temporal variation of these proportions makes it difficult to identify the species and populations that are most vulnerable. The magnitude of our mortality estimates suggest that cats are likely causing population declines for some species and in some regions. Threatened and endangered wildlife species on islands are most susceptible to the effects of cat predation, and this may also be true for vulnerable species in localized mainland areas [5] because small numbers of fatalities could cause significant population declines. Threatened species in close proximity to cat colonies—including managed TNR colonies [11] , [12] —face an especially high level of risk; therefore, cat colonies in such locations comprise a wildlife management priority. Claims that TNR colonies are effective in reducing cat populations, and, therefore, wildlife mortality, are not supported by peer-reviewed scientific studies [11] . Our estimates should alert policy makers and the general public about the large magnitude of wildlife mortality caused by free-ranging cats. Structured decisions about actions to reduce wildlife mortality require a quantitative evidence base. We provide evidence of large-scale cat predation impacts based on systematic analysis of multiple data sources. Future specific management decisions, both in the United States and globally, must be further informed by fine scale research that allows analysis of population responses to cats and assessment of the success of particular management actions. We are not suggesting that other anthropogenic threats that kill fewer individuals are biologically unimportant. Virtually nothing is known about the cumulative population impacts of multiple mortality sources. Furthermore, comparison of total mortality numbers has limited use for prioritization of risks and development of conservation objectives. Combining per species estimates of mortality with population size estimates will provide the greatest information about the risk of population-level impacts of cat predation. Although our results suggest that owned cats have relatively less impact than un-owned cats, owned cats still cause substantial wildlife mortality ( Table 2 ); simple solutions to reduce mortality caused by pets, such as limiting or preventing outdoor access, should be pursued. Efforts to better quantify and minimize mortality from all anthropogenic threats are needed to increase sustainability of wildlife populations. The magnitude of wildlife mortality caused by cats that we report here far exceeds all prior estimates. Available evidence suggests that mortality from cat predation is likely to be substantial in all parts of the world where free-ranging cats occur. This mortality is of particular concern within the context of steadily increasing populations of owned cats, the potential for increasing populations of un-owned cats [12] , and an increasing abundance of direct and indirect mortality sources that threaten wildlife in the United States and globally. Literature search We searched JSTOR, Google Scholar, and the Web of Science database (formerly ISI Web of Science) within the Web of Knowledge search engine published by Thomson Reuters to identify studies that document cat predation on birds and mammals. We initially focused this search on US studies, but due to a limited sample of these studies, we expanded the search to include predation research from other temperate regions. We also searched for studies providing estimates of cat population sizes at the scale of the contiguous United States and for US studies that estimate the proportion of owned cats with outdoor access and the proportion of cats that hunt wildlife. The search terms we used included: ‘domestic cat’ in combination with ‘predation,’ ‘prey,’ ‘diet,’ ‘food item’ and ‘mortality’; all previous terms with ‘domestic cat’ replaced by ‘ Felis catus ,’ ‘feral,’ ‘stray,’ ‘farm,’ ‘free-ranging,’ and ‘pet’; ‘trap-neuter-return colony’; ‘TNR colony’; and ‘cat predation’ in combination with ‘wildlife,’ ‘bird,’ ‘mammal,’ and ‘rodent’. We checked reference lists of articles to identify additional relevant studies. Lead authors of three studies were also contacted to enquire whether they knew of ongoing or completed unpublished studies of cat predation in the United States. Classification of cat ranging behaviour We grouped studies based on the ranging behaviour of cats investigated. We defined owned cats to include owned cats in both rural and urban areas that spend at least some time indoors and are also granted outdoor access. We defined un-owned cats to include all un-owned cats that spend all of their time outdoors. The un-owned cat group includes semi-feral cats that are sometimes considered pets (for example, farm/barn cats and strays that are fed by humans but not granted access to habitations), cats in subsidized (including TNR) colonies, and cats that are completely feral (that is, completely independent and rarely interacting with humans). We did not classify cats by landscape type or whether they receive food from humans because the amount of time cats spend outdoors is a major determinant of predation rates [33] , [34] and because predation is independent of whether cats are fed by humans [6] , [34] , [35] . Study inclusion criteria Studies were only included if: (1) they clearly reported cat ranging behaviour (that is, a description of whether cats were owned or un-owned and whether they were outdoor cats or indoor-outdoor cats), and (2) the group of cats investigated fit exclusively into one of the two groups we defined above (that is, we excluded studies that lumped owned and un-owned cats in a single predation rate estimate). For some studies, we extracted a portion of data that met these criteria but excluded other data from cats with unknown ranging behaviour. We only included mainland and large island (New Zealand and United Kingdom) predation studies, because cat predation on small islands is often exceptionally high [36] , [37] and focused on colony nesting seabirds [38] . We excluded studies from outside temperate regions and those with predation rate estimates based on fewer than 10 cats, <1 month of sampling, or on cats that were experimentally manipulated (for example, by fitting them with bells or behaviour altering bibs). We included studies that used cat owners’ records of prey returns, but we excluded those that asked owners to estimate past prey returns because such questionnaires may lead to bias in estimation of predation rates [39] . (For a list of all included and excluded studies, see Supplementary Table S1 ). Data extraction and standardization of predation rates Most studies report an estimate of cat predation rate (that is, daily, monthly or annual prey killed per cat) or present data that allowed us to calculate this rate. When studies only reported predation rate estimates for all wildlife combined, we calculated separate predation rates by extracting taxa-specific prey counts from tables or figures and multiplying the total predation rate by the proportion of prey items in each taxon. If taxa-specific counts were not provided, we directly contacted authors to obtain this information. For studies that presented low, medium and high estimates or low and high estimates, we used the medium and average values, respectively. For studies that presented more than one predation estimate for cats with similar ranging behaviour (for example, owned cats in rural and urban areas), we calculated the average predation rate. Nearly all studies of un-owned cats report numbers or frequencies of occurrence of different taxa in stomachs and/or scats. For studies reporting numbers of prey items, we estimated annual predation rates by assuming one stomach or scat sample represented a cat’s average daily prey intake (for example, an average of one prey item per stomach or scat=365 prey per cat per year). This assumption likely resulted in conservative estimates because cats generally digest prey within 12 h (ref. [28] 28) and can produce two or more scats each day [29] . For studies reporting occurrence frequencies of prey items, we assumed this proportion represented a cat’s average daily prey intake (for example, a 10% bird occurrence rate=0.1 bird per stomach or scat=36.5 birds per cat per year). This assumption results in coarse predation rate estimates, but estimates from this approach are even more conservative than those from the first assumption because many stomachs and scats undoubtedly included more than one bird or mammal. Predation rate estimates from many studies were based on continuous year-round sampling or multiple sampling occasions covering all seasons. However, seasonal coverage of some studies was incomplete. To generate full-year predation rate estimates in these cases, we adjusted partial-year predation estimates according to the average proportion of prey taken in each month as determined from year-round studies reporting monthly data (birds and mammals [8] , [33] , birds only [7] , [40] ). For partial-year estimates from the northern hemisphere, we offset monthly estimates from southern hemisphere studies by 6 months. The final annual predation rate estimates for all studies are presented in Supplementary Table S1 . The year-round studies we used represent different geographical regions (for birds—England, Kansas (US), Australia and New Zealand; for mammals—England and Australia) with varying climates and slightly varying seasonal patterns of predation. For both birds and mammals, averaging across full-year studies resulted in higher proportions of predation in the spring and summer compared with fall and winter, an expected pattern for much of the United States. The reference studies we used, therefore, provide a reasonable baseline for correcting to full-year mortality estimates. This approach greatly improves upon the assumption that mortality is negligible during the period of the year not covered by sampling. Quantification of annual mortality from cat predation We estimated wildlife mortality in the contiguous United States by multiplying data-derived probability distributions of predation rates by distributions of estimated cat abundance, following [41] . Quantification was conducted separately for owned and un-owned cats and for birds and mammals. As there was a relatively small sample of US studies that estimated predation rates ( n =14 and 10 for birds and mammals, respectively), we repeated calculations using predation rate distributions that were augmented with predation rates from Europe and all temperate zones. However, we only used studies from the contiguous United States to construct all other probability distributions (listed below). We estimated mortality using the following model of cat predation: where npc is the number of owned cats in the contiguous United States, pod is the proportion of owned cats granted outdoor access, pph is the proportion of outdoor owned cats that hunt wildlife, ppr is the annual predation rate by owned cats, cor is a correction factor to account for owned cats not returning all prey to owners, nfc is the number of un-owned cats in the contiguous United States, pfh is the proportion of un-owned cats that hunt wildlife, and fpr is the annual predation rate by un-owned cats. From the probability distribution of each parameter (see Table 1 and Supplementary Methods for details about the specific probability distributions used), we randomly drew one value and used the above formulas to calculate mortality. Random draws were made using distribution functions in Programme R (rnorm and runif commands for normal and uniform distributions, respectively). We conducted 10,000 random draws to estimate a potential range of annual predation on each wildlife taxa. For all analyses, we report median mortality estimates and lower and upper estimates bracketing the central 95% of values. Sensitivity analyses We used multiple linear regression analysis to assess how much variance in mortality estimates was explained by the probability distribution for each parameter. We treated total mortality estimates as the dependent variable ( n =10,000) and we defined a predictor variable for each parameter that consisted of the 10,000 randomly drawn values. We used adjusted R 2 values to interpret the percentage of variance explained by each parameter. How to cite this article: Loss S.R. et al . The impact of free-ranging domestic cats on wildlife of the United States. Nat. Commun. 4:1396 doi: 10.1038/ncomms2380 (2012).